Electric in-plane polarization in multiferroic CoFe2O4/BaTiO3nanocomposite tuned by magnetic fields Ferrimagnetic CoFe 2 O 4 nanopillars embedded in a ferroelectric BaTiO 3 matrix are an example for a two-phase magnetoelectrically coupled system. They operate at room temperature and are free of any resource-critical rare-earth element, which makes them interesting for potential applications. Prior studies succeeded in showing strain-mediated coupling between the two subsystems. In particular, the electric properties can be tuned by magnetic fields and the magnetic properties by electric fields. Here we take the analysis of the coupling to a new level utilizing soft X-ray absorption spectroscopy and its associated linear dichroism. We demonstrate that an in-plane magnetic field breaks the tetragonal symmetry of the (1,3)-type CoFe 2 O 4 /BaTiO 3 structures and discuss it in terms of off-diagonal magnetostrictive-piezoelectric coupling. This coupling creates staggered in-plane components of the electric polarization, which are stable even at magnetic remanence due to hysteretic behaviour of structural changes in the BaTiO 3 matrix. The competing mechanisms of clamping and relaxation effects are discussed in detail. Multiferroic materials showing both magnetic and electric ordering allow an additional degree of freedom in the design of actuators, transducers and storage devices and thus have attracted scientific interest from the technological perspective as well as from basic research [1] . Because the choice of single-phase multiferroic materials being suitable at room temperature is limited, the use of magnetoelectric two-phase composites has proven to be more promising [2] . Recently, even classic materials such as ferromagnetic Fe and ferroelectric BaTiO 3 (BTO) have been shown as potentially useful [3] . They reveal electric field-controllable magnetoelectric coupling via interfacial spin polarization of Ti 4+ . Research on core-shell nanoparticles had shown that the spin polarization of Ti 4+ at the interfaces between BTO and Fe and its oxides remains virtually negligible [4] . Hence, two-phase composites of a piezoelectric and a magnetostrictive phase, which can be magnetoelectrically coupled via stress mediation [5] , still remain favourites of the current discussion [6] . One of the prime candidates of such systems is the BTO/CoFe 2 O 4 (CFO) system. CFO is a ferrimagnet below T c =790 K with an inverse spinel structure that exhibits a remarkable magnetostriction of up to λ || ≈−2 × 10 −4 along the direction of the applied magnetic field (longitudinal magnetostriction) and ≈1 × 10 −4 for transverse magnetostriction at room temperature [7] . The strength of magnetostriction strongly depends on the cation distribution in CFO. The inverse spinel structure (space group Fd m ; no. 227) is a cubic crystal system, with oxide anions arranged in a cubic close-packed lattice and metal cations tetragonally or octahedrally surrounded by the oxygen. Each unit cell consists of 32 oxygen ions, 16 octahedral sites and 8 tetrahedral sites. For CFO, Fe 3+ ions occupy the tetrahedral sites and half of the octahedral sites, whereas Co 2+ ions are located at the remaining octahedral sites. Three crystallographic phases of BTO are ferroelectric: rhombohedral <190 K, orthorhombic for 190 K< T <278 K and tetragonal for 278 K< T <395 K. At higher temperatures, BTO is paraelectric. In this work, all measurements were performed at room temperature, where BTO has a tetragonal unit cell (space group P 4 mm ; no. 99) with the lattice parameters a = b =0.3992, nm and c =0.4036, nm. The occurence of the spontaneous electric polarization is connected to a displacement of the Ti 4+ ion along the crystallographic c axis and a sensitive charge hybridization of the 3 d states of the Ti cation with the 2 p states of the surrounding O anions. By density functional theory within the local spin density approximation, it has been shown that the off-centre displacement is connected to a substantial charge rearrangement changing the occupation of the , d xz , and d yz orbitals of Ti to slightly higher values at the expense of electron occupation of the d xy orbital of Ti and p orbitals of the oxygen ions located on the z axis yielding a destabilization of the centrosymmetric configuration [8] . On a macroscopic scale, piezoelectric coefficients of p || z ≈150 pm V −1 along the z axis and ≈−80 pm V −1 along x and y axis were found [9] . As previously shown [10] , structural compatibility of CFO with BTO allows growth of different two-phase heterostructures when using SrTiO 3 (STO) as a substrate. The resulting combination of magnetostrictive CFO with piezoelectric BTO presents an artificial multiferroic composite whose electric polarization P can by tuned by a magnetic field and whose magnetic properties can be altered by an electric field [11] , respectively, by strain mediation. In the literature (for example, Zheng et al. [10] ), multilayered (2,2)-structures of CFO and BTO are reported, as well as vertically aligned (1,3)-structures ( Fig. 1a ). The latter configuration minimizes clamping effects to the substrate that substantially reduce the possible structural deformations and is also used in this work. To achieve complete regularity of the nanopillar pattern, a recently experienced stencil-derived direct epitaxy technique [12] might eventually be chosen for pertinent applications. From application’s point of view, our quasi-two-dimensional assembly of nanopillars of CFO embedded in BTO as introduced by Zheng et al. [10] is a prototype system for electrically addressable magnetic data-storage devices working at room temperature. However, for all future applications, an understanding of the coupling mechanism between the two constituents is essential. Although in phase-field simulations, electrostriction (strain P 2 ) in BTO has often exclusively been taken into account [13] , piezoelectricity (strain P ) is rarely discussed [14] . 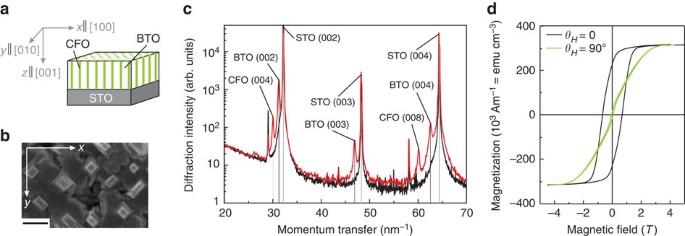Figure 1: Sample pre-characterization. (a) Illustration of nanopillar structure and introduction of sample coordinate system. Scale bar, 200 nm. (b) Scanning electron microscopy image of the sample corresponding to a top view on the nanopillar structure. (c) X-ray diffraction evidencing the strongly texturized growth and phase separation between BTO and CFO. The red line corresponds to the measurement of the sample in total, and the black line corresponds to the substrate only. (d) SQUID magnetometry at room temperature reveals the easy direction of magnetization along the sample normal. Figure 1: Sample pre-characterization. ( a ) Illustration of nanopillar structure and introduction of sample coordinate system. Scale bar, 200 nm. ( b ) Scanning electron microscopy image of the sample corresponding to a top view on the nanopillar structure. ( c ) X-ray diffraction evidencing the strongly texturized growth and phase separation between BTO and CFO. The red line corresponds to the measurement of the sample in total, and the black line corresponds to the substrate only. ( d ) SQUID magnetometry at room temperature reveals the easy direction of magnetization along the sample normal. Full size image In this work, hitherto neglected non-diagonal piezoelectricity components are taken into account for the first time. They are shown to be crucial for the observed changes in local charge symmetry and analysed to gain a more detailed understanding of the microscopic coupling effect between CFO and BTO. In this regard, the soft X-ray absorption spectroscopy and its associated circular and linear dichroism offer the unique possibility to study both spin and charge anisotropy element specifically. Thus, by applying magnetic fields, it is possible not only to measure the magnetic response of the CFO but also to monitor changes in the electronic structure of the BTO host matrix, especially the changes around the Ti 4+ ions as done in this work. Phase-separated growth and pre-characterization The sample was prepared by pulsed laser deposition from a target consisting of 65% BTO and 35% CFO. Details of the sample preparation can be found in the Methods section. A spontaneous phase separation between the BTO and CFO makes the growth of self-assembled CFO pillars in a BTO matrix possible. Scanning electron microscopy ( Fig. 1b ) images reveal a quasi-periodic assembly of CFO pillars with rectangular cross-sections, the mean edge-length in the sample plane being about 70 nm and the length around 400 nm. A scanning electron microscopy image over a large sample area is shown in Supplementary Fig. S1 . From atomic force microscopy, we found that the length of the CFO pillars is about 10% larger than the thickness of the BTO matrix. X-ray diffraction ( Fig. 1c ) shows a clear phase separation of the constituents and a (001) texture. For the crystallographic in-plane axes, we have CFO[010]||BTO[010]||STO[010] that have been chosen here as y axis and CFO[100]||BTO[100]||STO[100] that have been chosen as x axis. Please note, that the BTO/CFO interfaces at the sides of the nanopillars are {110}-type planes similarly as verified for the related BFO(=BiFeO 3 )/CFO system [15] . To avoid the impression that the in-plane crystallographic axes of the CFO nanopillars could be rotated with respect to the ones of BTO, the unit cell orientation of CFO is depicted in the schematic figures in this work. The in-plane mosaicity is well <1° for both CFO and BTO as discussed in the Supplementary Methods . The corresponding X-ray diffraction peaks are shown in Supplementary Fig. S2 , and the results are summarized in Supplementary Table S1 . This high quality of epitaxial growth is crucial for the proper analysis of the X-ray absorption spectroscopy measurements. Magnetometry using a superconducting quantum interference device (SQUID) clearly shows that the easy axis of magnetization points along z as expected because of the shape anisotropy of the nanopillars ( Fig. 1d ). The magnetization is normalized to the CFO fraction in the sample, and its saturated value of M s =(3.15±0.4) × 10 5 Am −1 is in agreement with the one reported in the literature [10] . The anisotropy field can be estimated by linear extrapolation of the field-dependent magnetization along the hard axis yielding about (2.5±0.5) T. Calculating the shape anisotropy within the Stoner Wohlfarth model for a slender prolate ellipsoid [16] with an aspect ratio of about r =5.7, the shape anisotropy field of the nanopillars amounts to μ 0 M s (1+1/ r 2 [1−ln(2 r )])/2≈0.19 T in agreement to the value reported by Zheng et al. [10] who explained the difference between the estimated anisotropy from experimental magnetometry data and the calculated shape anisotropy due to demagnetizing fields by the occurence of the magnetoelastic coupling. Crystal field parameters of BTO in magnetic remanence Soft X-ray absorption spectra were taken at the L 3,2 absorption edges of Ti and Co at which electrons are excited from the 2 p 3/2 and 2 p 1/2 core levels into the 3 d states and at the M 5,4 absorption edges (3 d 5/2 and 3 d 3/2 into the 4 f states) of Ba, respectively. An overview spectrum over the elements is presented in Supplementary Fig. S3 . For linearly polarized light, the electric field vector of the X-rays acts like a search light for the unoccupied density of states. As an example, let us consider the d orbital: If the electric field vector is parallel to the z axis, the absorption is maximum, whereas for the case of the electric field vector lying in the xy plane or including any non-vanishing angle with the z axis, the absorption will be lower. In Fig. 2 , the relation between the X-ray absorption at the Ti L 3 edge and the 3 d orbitals is depicted: the two absorption maxima occur due to electronic transitions towards the lower-energetic d xz , d yz and d xy orbitals on the one hand and the higher-energetic d and d on the other hand. Because of hybridization effects, for example, orbitals pointing towards the oxygen ligands yield broader absorption lines in the absorption spectrum. The additional energy splitting due to the Ti displacement is too small to be directly visible in the absorption spectrum. However, it can be analysed by measuring the dichroism between two different directions of linear polarization. For a quantitative analysis of the X-ray linear dichroism (XLD), the sample has been measured under grazing incidence ( θ k =60°), so the main component of the electric field vector of the X-rays is either perpendicular to the z axis (vertical polarization) or along the z axis (horizontal polarization) as sketched in Supplementary Fig. S4 . Because the angle of incident X-ray cannot be θ k =90° for technical reasons, the spectral intensities have been recalculated according to our measurement geometry to obtain the full linear dichroism. As also the in-plane component of the wave vector k of incident X-rays may be important when analysing the XLD (ref. 17 ), k was kept in the yz plane for all measurements presented here. The same holds for the external magnetic field. Measurements in normal incidence ( θ k =0) do not require any correction. In that case, the electric field vector of the vertically and horizontally polarized X-rays is along the x and y direction, respectively. Details on both exact measurement geometry and corrections, respectively, can be found in the Methods section and Supplementary Fig. S4 . 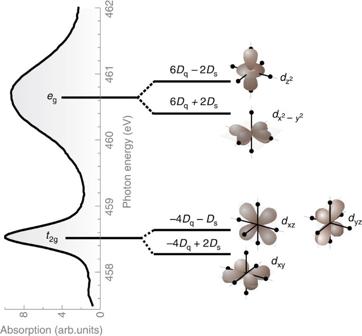Figure 2: Relating XAS and atomic orbitals. The soft X-ray absorption spectrum at theL3edge of Ti (left) is related to the energy levels of the Ti ion in the crystal field for positive values of 10Dqand negative values ofDs. (Dtis neglected.) In the tetragonal phase of BTO, the energy levels of the cubicegandt2gstates further split into sublevels. The energy scale for this splitting is stretched. Figure 2: Relating XAS and atomic orbitals. The soft X-ray absorption spectrum at the L 3 edge of Ti (left) is related to the energy levels of the Ti ion in the crystal field for positive values of 10 D q and negative values of D s . ( D t is neglected.) In the tetragonal phase of BTO, the energy levels of the cubic e g and t 2g states further split into sublevels. The energy scale for this splitting is stretched. Full size image In Fig. 3 , the experimental soft X-ray absorption near-edge structure (XANES) and the associated XLD of Ti in magnetic remanence after magnetizing along the z direction ( μ 0 H =3 T) are compared with charge-transfer multiplet calculations using the CTM4XAS program [18] . The following discussion of the influence of the Ti 4+ ion displacement on the X-ray absorption spectra is based on crystal field parameters. A short introduction to crystal field theory and its connection to XAS can be found, for example, in the work of de Groot [19] . We would like to mention that the value of the crystal field parameter 10 D q denotes the energy splitting between the t 2g and e g states in a cubic symmetry as depicted in Fig. 2 , whereas D s takes into account the deviation from a cubic symmetry including the displacement of the Ti 4+ ion. The best fit to experimental data was obtained for the crystal field parameters 10 D q =2.0 eV, in agreement with de Groot et al. [20] and Chassé et al. [21] , and D s =−0.04 eV. Note that the XANES is not very sensitive to changes of D s , whereas the XLD strongly depends on this value and vanishes for D s =0. The negative value of D s ensures the correct energy splitting of t 2g and e g states into sublevels in accordance with band structure calculations reported in the literature for tetragonal BTO [8] . In that reference, Filippetti and Hill calculated the density of states for Ti 4+ in BTO for a cubic and tetragonal unit cell by a plane-wave pseudopotential implementation of density functional theory within the local spin density approximation (LSDA) [22] , and assigned it to atomic orbitals. In the tetragonal phase, the displacement of the Ti 4+ from its centrosymmetric position along the z direction yields a splitting between the d xy orbital and the orbitals with a significant z component, that is, d xz and d yz , which are at higher energies. From the view of crystal field parameters, this is equivalent to the introduction of a negative value of D s as depicted in Fig. 2 . Note that from the parameter D s , the geometric structure cannot be deduced directly [23] . Here the negative value of D s is associated with an elongation of the BTO unit cell along the z direction. This is in agreement to XRD data revealing that the the elongated axis of the tetragonal BTO is parallel to z ( cf . Fig. 1c ). Using these values for the crystal field, not only the spectral shape of XANES and XLD are reasonably reproduced by our simulations but also the XLD amplitude fits well. Thus, one can conclude that the electric polarization in the sample points along z as it was assumed in the simulation. 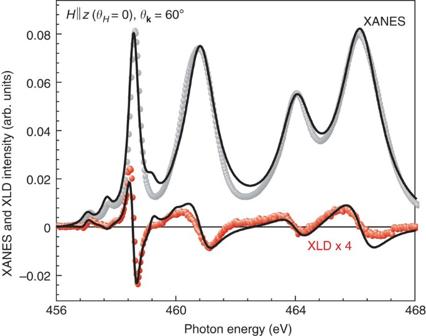Figure 3: Simulation and experimental data. Soft XANES and its associated XLD from experiment (symbols) and simulation (lines). Measurements were performed in magnetic remanence after magnetically saturating the sample along thezdirection (θH=0) under grazing incidence (θk=60°) and were corrected for the angular misalignment to obtain full dichroism. Figure 3: Simulation and experimental data. Soft XANES and its associated XLD from experiment (symbols) and simulation (lines). Measurements were performed in magnetic remanence after magnetically saturating the sample along the z direction ( θ H =0) under grazing incidence ( θ k =60°) and were corrected for the angular misalignment to obtain full dichroism. Full size image Electric in-plane polarization in magnetic remanence Measuring the soft X-ray absorption in magnetic remanence after magnetizing along z ( θ H =0, μ 0 H =3 T) in normal incidence, that is, with the electric field vector of incident soft X-rays perpendicular to z for both horizontal and vertical polarization, does not give rise to a dichroic signal as can be seen in Fig. 4a , left panel. This is because of the fact that the d , d and d xy , and the sum of the energetically degenerated d xz and d yz , have the same 90° symmetry in the xy plane as the electric field vectors for horizontally and vertically polarized X-rays probing these orbitals. Let us consider the 90° symmetry of the BTO orbitals observed after magnetizing along the z direction in terms of the ferroelectric polarization. In a simple picture, the magnetic field gives rise to a contraction of the CFO nanopillars ( λ || <0). Because of Poisson’s law, the pillars have the tendency to expand in the xy plane ( >0). Close to the substrate, this expansion is hindered by clamping effects through the substrate, whereas near the surface, they have the possibility to expand in both x and y directions by compressing the BTO matrix. By virtue of the non-vanishing piezoelectric shear coefficients [24] , this gives rise to the evolution of in-plane components P x and P y of the electric polarization, as schematically shown in Fig. 4b . In this geometry, x and y directions are equivalent in agreement to the 90° in-plane symmetry obtained in the experiment (| P x |=| P y |). 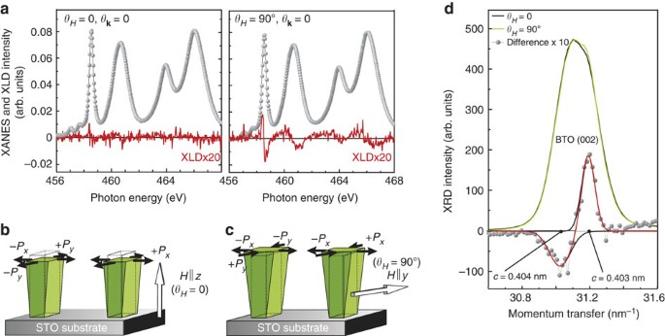Figure 4: Experimental soft X-ray absorption and X-ray diffraction in magnetic remanence. (a) Soft XANES and XLD in normal incidence (θk=0) in magnetic remanence after magnetically saturating the sample along thezdirection (θH=0) andydirection (θH=90°), respectively. (b,c) Illustration of different experimental geometries and (deformed) shapes of CFO nanopillars’ unit cells with apical polarization vectors of the BTO environment ±Px,y. (d) X-ray diffraction at the BTO (002) peak in magnetic remanence after magnetically saturating the sample along thezdirection (black line,θH=0) andydirection (green line,θH=90°), respectively. Symbols refer to the difference of the two diffraction signals (enlarged by a factor of 10), and the red line refers to a fit using two Gaussian distributions. Formally, this can be written as Figure 4: Experimental soft X-ray absorption and X-ray diffraction in magnetic remanence. ( a ) Soft XANES and XLD in normal incidence ( θ k =0) in magnetic remanence after magnetically saturating the sample along the z direction ( θ H =0) and y direction ( θ H =90°), respectively. ( b , c ) Illustration of different experimental geometries and (deformed) shapes of CFO nanopillars’ unit cells with apical polarization vectors of the BTO environment ± P x,y . ( d ) X-ray diffraction at the BTO (002) peak in magnetic remanence after magnetically saturating the sample along the z direction (black line, θ H =0) and y direction (green line, θ H =90°), respectively. Symbols refer to the difference of the two diffraction signals (enlarged by a factor of 10), and the red line refers to a fit using two Gaussian distributions. Full size image where d 15 is the decisive and quite sizable off-diagonal piezoelectric coefficient [24] , and σ 13 and σ 23 are components of the stress tensor causing the shear in xz and yz planes, respectively. It should be emphasized, again, that the non-zero shear stress components σ 13 and σ 23 are most important consequences of the nanopillar clamping at the STO substrate ( Fig. 4b ). The quadratic deformation of the CFO unit cell cross-sections is by symmetry characterized by | σ 13 |=| σ 23 |. In contrast, application of the external magnetic field in the sample plane, for example, along the y direction ( θ H =90°, μ 0 H =3 T), breaks this symmetry because the nanopillars contract in y direction and expand in x (and z ) direction yielding a rectangular deformation of the unit cell cross-sections of the nanopillars with | σ 13 |≠| σ 23 |. This leads to a compression of the BTO along the x direction only and to directly opposed in-plane polarization components as sketched in Fig. 4c and in more detail in Supplementary Fig. S5 . As a consequence, a measurable XLD signal evolves under normal incidence of the X-rays ( Fig. 4a , right panel), reflecting the spatial in-plane anisotropy of the electric polarization (| P x |≠| P y |). It can be switched on and off by application of an in-plane external magnetic field or a magnetic field perpendicular to the sample plane, respectively, and is stable in magnetic remanence. By comparison with the XLD presented in Fig. 3 , its amplitude clearly exceeds the value of 0.01 P z estimated in the Supplementary Methods . This may be due to a reduced value of P z because we did not apply an electric field to obtain the XLD presented in Fig. 3 . However, the large in-plane XLD signal indicates an induced charge anisotropy on a macroscopic length scale that is not restricted to the CFO/BTO interface. Comparing the sign of the XLD signals shown in Figs 3 and 4a , respectively, one can conclude that the more elongated in-plane axis of BTO after magnetizing along the y direction is indeed the y axis supporting the model presented above. From our measurements, one can conclude that an in-plane component of the electric polarization of the BTO can be tuned by application of an external magnetic field. This change of the electric polarization towards x and y directions [24] is quite significant for BTO. It can be modelled within the Ginzburg Landau theory [25] and has been assigned to the vicinity of the phase transition from the tetragonal phase at room temperature to the orthorhombic phase of BTO at about 278 K (ref. 26 ). To confirm that the XLD is caused by an in-plane component of the electric polarization due to different remanent mechanical stresses on the BTO matrix, we performed X-ray diffraction (XRD) measurements under the same conditions as for the previous XLD measurements. That is, XRD scans were taken in magnetic remanence after application of a magnetic field ( μ 0 H =3 T) either along the z direction or along the y direction. We focused on the (00L) reflections, that is (002) for BTO and STO substrate and (004) for CFO ( cf . Supplementary Fig. S2 ). The diffraction peak for BTO is presented in Fig. 4d . After magnetizing along the z direction, the BTO (002) peak is asymmetric that is related to the gradient of the magnetostriction of CFO due to the clamping to the substrate as depicted in Fig. 4b . The position of the peak maximum corresponds to a lattice constant of c ≈0.404 nm in agreement to the expected bulk value for the long axis of the BTO unit cell. Applying the magnetic field in the sample plane yields the evolution of a second peak at higher momenta corresponding to a reduced lattice constant of about 0.402 nm (not shown here). After removing the magnetic field, the second peak is smaller, but still visible, and corresponds to an intermediate reduced lattice constant c ′≈0.403 nm ( Fig. 4d ). This behaviour can be understood as the response of the matrix to different in-plane stresses by the CFO pillars. When the external magnetic field was applied perpendicularly to the sample plane, we have a compression of the BTO in both x and y directions as explained above, reducing the lattice constants a and b . The lattice constant c will be an equilibrium value determined by two competing mechanisms: on the one hand, the unit cell volume should be conserved, which favours an expansion of the c axis, and on the other hand, the BTO is coupled to the CFO pillars, which shows a contraction along that direction. This competition can also yield the asymmetric line shape of the BTO diffraction peak obtained here because it is reasonable that close to the BTO/CFO interface, the coupling between the constituents is dominant, whereas it is weaker at larger distances from the interface. When the sample is magnetized in-plane along the y direction, the BTO matrix is allowed to expand in this direction. To conserve the unit cell volume, BTO should exhibit a reduced value of the c axis. However, because CFO shows a lattice expansion in this case, we end up with two competing contributions again. But this time, the positive magnetostriction of CFO along the z axis for H || y is only half the absolute value of the magnetostriction for H || z because the longitudinal magnetostriction is up to λ || ≈−2 × 10 −4 , whereas the transverse magnetostriction is ≈1 × 10 −4 (ref. 7 ). Therefore, the structural relaxation of the BTO when distancing the BTO/CFO interface may appear sooner. In addition, especially at the surface of the sample where clamping is negligible, the in-plane contraction of the nanopillars along y and, consequently, the expansion of the BTO along y may be significant. That means, parts of the sample have different in-plane lattice constants, a < b , and a reduced c lattice constant compared with the bulk value as obtained in the X-ray diffraction data. As already mentioned above, the phase-transition temperature from the tetragonal phase to the orthorhombic phase of BTO (at 278 K) is quite close, facilitating the occurence of in-plane components of the electric polarization as well as structural deformations. Similarly to the broad thermal hysteresis of the BTO structure (about 10 K (ref. 26 )), a field-dependent hysteretic behaviour of the structure as evidenced here appears reasonable. The obtained distortion of the former tetragonal unit cell in combination with the shear forces depicted in Fig. 4c makes it possible to tune an in-plane component of the electric polarization of the BTO host matrix. Magnetic field dependence of induced electric polarization To prove that there is a direct coupling between CFO and BTO, the XLD signals at the Ti ions have been measured as a function of external magnetic field in two different geometries: with the main component of the magnetic field either along the z axis or perpendicular, that is, along the y axis ( Supplementary Fig. S4 ). The resulting Ti XLD asymmetries, that is, the XLD divided by the sum of absorption spectra measured with vertical and horizontal polarization of X-rays ( I ver − I hor )/( I ver + I hor ), are plotted in Fig. 5a . For a reasonable analysis of the small dichroic signals, only amplitudes of the XLD asymmetry averaged over both absorption edges are presented, as shown in Supplementary Fig. S6 and discussed in the Methods section. 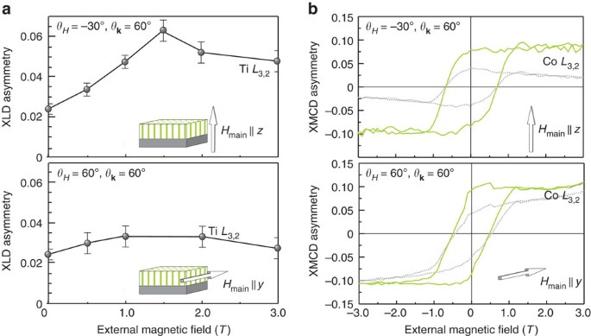Figure 5: Changing the Ti XLD by external magnetic fields. (a) Field-dependent soft XLD at the TiL3,2absorption edges measured under grazing incidence (θk=60°) for different directions of the magnetic field with the main componentHmaineither parallel tozor perpendicular toz. Error bars are estimated by comparison of 2–5 pairs of spectra to extract the XLD asymmetry and slight energy variation. (b) Field-dependent soft X-ray magnetic circular dichroism at the CoL3absorption edge as a measure of magnetization for the same geometries as ina. Grey dotted lines correspond to raw data, and green solid lines correspond to the XMCD signal after elimination of field-dependent rotation of the magnetization, assuming an anisotropy field of 2.5 T. Figure 5: Changing the Ti XLD by external magnetic fields. ( a ) Field-dependent soft XLD at the Ti L 3,2 absorption edges measured under grazing incidence ( θ k =60°) for different directions of the magnetic field with the main component H main either parallel to z or perpendicular to z . Error bars are estimated by comparison of 2–5 pairs of spectra to extract the XLD asymmetry and slight energy variation. ( b ) Field-dependent soft X-ray magnetic circular dichroism at the Co L 3 absorption edge as a measure of magnetization for the same geometries as in a . Grey dotted lines correspond to raw data, and green solid lines correspond to the XMCD signal after elimination of field-dependent rotation of the magnetization, assuming an anisotropy field of 2.5 T. Full size image We start the discussion with the common geometry of the magnetic field’s main component applied parallel to the long axis of the CFO nanopillars, that is, the z axis. The XLD of the Ti ions is increasing with increasing field by a factor of 3 to about 6.5% at an external magnetic field of 1.5 T. For higher external magnetic fields, a slight decrease is obtained, and the XLD is asymptotically approaching a value of about 5% for higher fields. This decrease is due to the fact that in our measurement geometry, the magnetic field could not be applied exactly parallel or perpendicular to the CFO nanopillars. As at about 1.5 T the CFO saturates, the effect of pulling the magnetization from its easy direction towards the direction of the external magnetic field significantly influences the field dependence of the XLD. In Fig. 5b , the raw data of the field-dependent magnetization are shown that exhibit an additional linear slope of the signal (grey dotted lines). This slope can be easily eliminated (green solid lines) by correcting the different angles between magnetization and external magnetic field, assuming an effective anisotropy field of 2.5 T in agreement to the anisotropy estimated by extrapolating SQUID magnetometry data, as discussed in the Supplementary Methods and sketched in Supplementary Fig. S7 . The comparison of the Ti XLD and the Co X-ray magnetic circular dichroism (XMCD) as a measure of the magnetization clearly evidences the correlation between these two values. As the XLD is a measure of the anisotropy of electronic states, it indicates on a microscopic scale the modification of the electric polarization of BTO by a magnetic field. When the external magnetic field is applied with its main component in-plane, the change of the XLD is quite small and increases from 2.2 to 3.5% with increasing field. This corresponds to our findings presented above: when the magnetic field is applied in-plane, that is, along the y direction, the CFO contracts in this direction, the surrounding BTO is allowed to expand while the c lattice parameter in z direction is slightly smaller, reducing the tetragonal distortion and the electric polarization along z consequently. This corresponds to a reduced XLD signal. In x direction, the BTO is compressed as for the case of a magnetic field applied along the z direction, yielding an enhanced XLD. On average, a slightly enhanced XLD is obtained. We conclude that the observed magnetic field dependences within our model clearly prove the direct coupling between the CFO nanopillars and the BTO matrix. The possibility of tuning the electric polarization of the BTO matrix hosting CFO nanopillars by an external magnetic field has been evidenced on a microsopic scale by correlating the charge anisotropies of the Ti ions (measured by XLD) with the spin anisotropies of Co ions (measured by XMCD). Although the electric polarization of the BTO matrix spontaneously points along the z direction in the as-grown state, it achieves shear stress-induced transverse components ± P x and ± P y , both under out-of-plane and in-plane magnetic fields. Field-induced quadratic and rectangular deformations, respectively, of the CFO unit cell cross-sections give rise to characteristic staggered modulations of the in-plane component of the electric polarization in BTO, reflecting the quasi-periodic distribution of the nanopillars and their deformation patterns. This has been verified by the spatial anisotropy of the averaged Ti XLD. The in-plane components of the electric polarization are still observed in magnetic remanence and are accompanied by a hysteretic behaviour in structural changes of BTO. The observed coupling yields a sizeable effect on the averaged electronic structure of BTO, much too large to be assigned to an interfacial effect like a charge transfer between BTO and CFO and a spin coupling between the polarization of Ti 4+ in BTO and Fe ions in CFO as in the work of Valencia et al. [3] Thus, the effect in the electric in-plane polarization of BTO obtained in this work extends over a large area. Under the constraint of completely regular arrays of CFO nanopillars [12] , one might even envisage data-storage concepts by encoding the local polarization patterns of single nanopillars ( Fig. 4c ) via external current-controlled local magnetic fields H x or H y . Sample preparation The sample was prepared by pulsed laser deposition from a commercially available target (Kurt J. Lesker company) containing 65 mol% BTO and 35 mol% CFO. Ultraviolet radiation was provided by a 248 nm KrF excimer laser (Lambda Physik) with a laser fluence of about 1 J cm −2 and a pulse repetition rate of 10 Hz. The 400 nm thick film was grown on STO(001)-oriented single-crystal substrate (CrysTec GmbH), which was kept at 950 °C during the growth in an oxygen atmosphere at 15 Pa (=0.15 mbar). A scanning electron microscopy image of a large area of the sample is shown in Supplementary Fig. S1 , revealing that the CFO nanopillars are quite homogeneously spread over the whole sample. The topography of the sample was investigated by atomic force microscopy and was found to show maximum variations in height of 10%, that is, about 40 nm. Sample pre-characterization by magnetometry and diffraction methods Magnetometry measurements were performed at 300 K using a commercial SQUID MPMS from Quantum Design providing magnetic fields up to ±5 T. The texturized growth was confirmed in conventional θ –2 θ geometry on a Philips PW 1730 diffractometer using Cu K α radiation at the University of Duisburg-Essen. For a more detailed analysis of the in-plane crystal order, X-ray diffraction has been carried out at the Helmholtz Center Berlin (HZB) on a conventional laboratory four-circle X-ray diffractometer using Mo K α radiation. Soft X-ray absorption spectroscopy For soft X-ray absorption experiments, the high-field endstation at beamline UE46-PGM1 of the HZB has been used at the HZB-BESSYII synchrotron radiation source. This endstation offers an in-plane rotable field up to ±6 T, and the beamline is well suited for the soft X-ray range with variable polarization, for example, linearly polarized light with the electric field vector lying either horizontal or vertical, as well as circularly polarized light. The measurement geometries are schematically shown in Supplementary Figs S4 and S7 . All measurements presented here were performed in total electron yield (TEY) mode by measuring the sample drain current at room temperature where BTO exhibits its tetragonal phase. Before the measurements, the time-dependent stability of the TEY has been monitored to exclude the occurrence of charging effects. Elemental analysis An additional chemical overview of the elements expected in the BTO/CFO sample, that is, Ba, Ti, O, Co and Fe, is given by the soft X-ray absorption spectra shown in Supplementary Fig. S3 . As the spectra were obtained in the TEY mode by measuring the sample drain current, which is very surface sensitive due to the small electron escape depth of a few nanometres, no signal from the STO substrate can be detected through the 400-nm thick BTO/CFO composite film. This ensures a reliable analysis also for the case of Ti, which is present in both STO substrate and BTO matrix. In Supplementary Fig. S3 , the soft XANES and its XLD are plotted for the elements. Here we present the measured TEY normalized to the incoming photon intensity without any background removal or any further treatment. The spectra were measured under grazing X-ray incidence ( θ k =60°) without a magnetic field applied, and the XLD reflects the charge anisotropy. For BTO, a clear XLD signal could be obtained at the Ti L 3,2 and Ba M 5,4 absorption edges, respectively. At the oxygen K edge, only a small dichroism could be obtained after measuring a smaller energy range with higher resolution. However, because oxygen is present in both BTO and CFO, an analysis of the XLD seems ambiguous. From the CFO nanopillars, a clear XLD signal is visible at both Fe and Co L 3,2 absorption edges. Soft XLD Soft X-ray absorption spectra have been measured under normal or grazing incidence as depicted in Supplementary Fig. S3 . In the former case, the electric field vector of the soft X-rays propagating along z is parallel to the x axis, and for horizontal polarization, it is parallel to the y axis. The linear dichroism obtained in this geometry reflects the charge anisotropy between x and y direction in the sample. To obtain the spectra in magnetic remanence shown in Fig. 5 of the main text, the magnetic field was applied either along z before the measurement or the sample was rotated by 90° around the x axis, the magnetic field was applied in y direction and the sample was rotated back to the former position after removal of the magnetic field. For grazing incidence, some corrections have to be done to overcome the angular misalignment. As can be seen in Supplementary Fig. S4b , the electric field vector for vertical polarization is again parallel to the x axis. For horizontal polarization, the electric field vector includes an angle θ −90°=30° with the z axis. Thus, the spectrum contains not only the pure spectrum of the electronic structure parallel to z but also a contribution of the electronic structure parallel to y . For the sake of simplification, the electric field vector components yielding spectra of the electronic structure along x and y are denoted in contrast to E || z . The related absorption intensities that are proportional to the electric field vector squared are denoted and I || z , respectively. Hence, the measured dichroism can be deduced as follows: That means, the dichroism obtained by simply subtracting the spectrum measured with horizontal polarization from the one measured with vertical polarization is smaller by a factor of , with respect to the real linear dichroism between the two directions along z and perpendicular to z , respectively. As a consequence, the linear dichroism measured under grazing incidence has been multiplied by . Note that for the case of an distorted BTO unit cell with the electric polarization not pointing along the z direction, the correction factor is larger. In our work, in some cases an in-plane component of the BTO electric polarization evolves as discussed in the main text. As the in-plane component cannot be quantified, we restrict to the correction presented above. In the unlikely case of a pure in-plane electric polarization of the BTO (with a fourfold symmetry), this procedure would underestimate the XLD by a factor of 2. The XLD asymmetries for Ti, Co and Ba are shown in Supplementary Fig. S6 for different magnetic fields. The XLD asymmetry refers to the difference between the absorption measured with either horizontal or vertical polarization of X-rays divided by the sum of the absorption measured with the two different polarizations, ( I ver − I hor )/( I ver + I hor ). This value is useful because it does not depend on the number of unoccupied final states but reflects changes in the polarization per unoccupied d state. It can clearly be seen that at the Co and Ba sites, only small magnetic field-induced changes occur, whereas at the Ti sites, the changes are significant. For a quantification of the XLD from measured spectra, the XLD amplitude has been analysed at various energies to minimize the error caused by noise. These XLD amplitudes used here are depicted in Supplementary Fig. S6 for the case of Ti. To obtain the averaged XLD, not only the occupation numbers for the initial states are taken into account, but also for the different t 2g and e g -like final d states. The Ti 4+ ion is characterized by totally empty d states; only a small fraction of the d states is occupied via hybridization with the electronic states of the surrounding oxygen atoms. Neglecting this hybridization effect yields fractions of 3/5 t 2g and 2/5 e g states resulting in , and for the XLD asymmetry, I (Ti)=( a + b )/3+(2 c +2 d )/3 with a–d being defined as sketched in Supplementary Fig. S6 (left). X-ray diffraction using synchrotron radiation X-ray diffraction measurements beyond the structural pre-characterization using a conventional laboratory X-ray source have been performed at the MAGS endstation of the 7T-MPW beamline at the HZB-BESSYII synchrotron radiation source. This endstation is composed of a Huber 5021 six-circle diffractometer and offers the possibility to apply magnetic fields up to ±5 T perpendicular to the scattering plane. Simulations Simulations were performed using the CTM4XAS charge-transfer multiplet software. This semi-empirical program is based on a Hartree–Fock method corrected for correlation effects to solve the atomic Hamiltonian [27] . It includes the core and valence spin-orbit coupling, the core-valence two-electron integrals (multiplet effects) and the effects of strong correlations within the charge-transfer model. In the case of metal ions in oxidic environment, this approach is known to give reliable results. More details about the program and some examples of applications can be found, for example, in Stavitski and de Groot [18] and de Groot et al. [28] To simulate the experimental data, the Slater integrals have been reduced to 0.81, and an individual Lorentzian peak broadening for the four peaks has been included similar to other reported values [20] . The peaks have been broadened by 0.17 eV; additional broadenings have been included for the peaks number 2–4: 0.62 eV for the second peak, 0.65 eV for the third peak and 0.80 eV for the fourth peak. Instrumental broadening was taken into account by an additional Gaussian broadening of 0.05 eV. For the case of XMCD measured at the Co L 3,2 absorption edges, the simulations can also be used to analyse possible cation disorder in CFO. However, comparison of our experimental data with simulated spectra of Co 2+ and Co 3+ as presented in Supplementary Fig. S8 clearly indicates that the majority of Co ions is in the 2+ state as expected for CFO. How to cite this article: Schmitz-Antoniak, C. et al. Electric in-plane polarization in multiferroic CoFe 2 O 4 /BaTiO 3 nanocomposite tuned by magnetic fields. Nat. Commun. 4:2051 doi: 10.1038/ncomms3051 (2013).